Network modularity reveals critical scales for connectivity in ecology and evolution For nearly a century, biologists have emphasized the profound importance of spatial scale for ecology, evolution and conservation. Nonetheless, objectively identifying critical scales has proven incredibly challenging. Here we extend new techniques from physics and social sciences that estimate modularity on networks to identify critical scales for movement and gene flow in animals. Using four species that vary widely in dispersal ability and include both mark-recapture and population genetic data, we identify significant modularity in three species, two of which cannot be explained by geographic distance alone. Importantly, the inclusion of modularity in connectivity and population viability assessments alters conclusions regarding patch importance to connectivity and suggests higher metapopulation viability than when ignoring this hidden spatial scale. We argue that network modularity reveals critical meso-scales that are probably common in populations, providing a powerful means of identifying fundamental scales for biology and for conservation strategies aimed at recovering imperilled species. Many ecological and evolutionary processes are inherently spatial, occurring at scales from millimetres to continents [1] , [2] . As a result, spatial scale can profoundly influence our understanding of these processes, altering conclusions regarding behaviour, population viability, species interactions and evolutionary dynamics [3] , [4] , [5] , [6] . Of great interest are critical (or characteristic) scales—spatial scales that govern the dynamics of key ecological and evolutionary processes [7] , [8] . Despite the significance of spatial scale, objectively identifying critical scales has been exceedingly difficult [3] , [9] . Consequently, our understanding of scale has been largely driven by patch-based [10] (or island-based [11] ) or larger landscape (summarized across all locations or patches in a pre-defined region) paradigms [8] , neither of which are typically defined by the key process of movement. Integrating the concept of modularity from physics [12] , cellular and molecular biology [13] , and social sciences [14] has the potential to fill this conceptual gap and objectively identify critical scales for populations [15] . In population biology, spatial modularity occurs where habitat patches (or local populations) are tightly connected to other patches through movement of individuals or their alleles but only weakly connected to the remaining patches in the landscape [15] . In doing so, spatial modularity provides a formal description of the functional aggregation of populations, identifies a potentially critical scale for ecological and evolutionary dynamics (for example, a relevant ‘management unit’ [9] ) and emphasizes the roles of patches in landscape connectivity based on movement within and between modules [15] , [16] . The emergence of modularity is crucial for population biology because several models suggest that such a structure can greatly influence dynamics [17] , [18] , [19] . Holt [19] catalysed this interest in the context of island biogeography by suggesting that internal island dynamics (for example, rescue effects [20] ) reduced extinction risk of populations, leading to altered predictions for biodiversity on islands; such internal dynamics are analogous to dynamics that may arise within modules. Similarly, a recent metapopulation model contrasting gradients of non-modular and modular metapopulations found that the most persistent metapopulations were those that were most modular [18] . Although theory suggests that modularity is highly relevant to spatial dynamics, the empirical application of modularity concepts to spatial ecology and evolution has been scarce. Recent algorithms from statistical physics and social sciences may help overcome these challenges while honouring complex dynamics that may arise in assessments of connectivity and critical spatial scales, such as highly directional movement [21] , spatial variation in the resolution of critical scales (that is, non-stationarity [22] ) and effects of scale beyond geographic distance alone [23] . Using four examples that vary in spatio-temporal scale regarding movement and gene flow, here we illustrate how the modularity concept can be applied to identify critical scales through the use of network analysis [12] . We quantify the extent to which populations are modular, reveal the spatial and non-spatial components of modularity and illustrate how module identification alters conclusions regarding connectivity and metapopulation persistence. We find significant modularity in the movement and gene flow of three of the four species, two of which cannot be explained by geographic distance alone. Furthermore, incorporating modularity into connectivity and population viability assessments alters conclusions regarding patch importance to connectivity and suggests higher metapopulation viability than when ignoring this hidden spatial scale. Revealing modularity in spatial networks We estimated modularity in two mark-recapture datasets that span several orders of spatial magnitude: movements of the cactus bug ( Chelinidea vittiger ) on patchy Opuntia cactus and breeding-season movements of the Everglades snail kite ( Rostrhamus sociabilis plumbeus ) among wetlands [21] . We also estimated modularity from genetic data on breeding aggregations of the bullfrog ( Rana catesbeiana ) [24] and among core populations of black bears ( Ursus americanus floridanus ) in Florida [25] . Based on the movement biology of each species, we expected that modularity should be weak in the Everglades snail kite and black bear because of frequently observed long-distance movements [26] , [27] , yet strong in the cactus bug and bullfrog because observed movements tend to be more localized [28] , [29] . We first assessed modularity by using extensions of the Newman–Girvan algorithm from statistical physics [30] that account for weighted (non-binary), directed network data where migration rates may differ. We find that three of the four examples exhibit significant spatial modularity based on generalized linear models testing for within versus between-module movement and gene flow (see Fig. 1a ; Supplementary Fig. S1 for assessments of this statistical test), with only the black bear showing no significant modularity ( Supplementary Table S1 ). However, modules showed a strong spatial signature, where patches within the same modules tended to be in close geographic proximity. Because movement of individuals and shared alleles are dependent on the distance between patches ( Fig. 1b ), geographic distance is a key (yet implicit) component of modularity on spatial networks and may confound our understanding of the mechanisms generating such structure. All empirical examples of modularity in ecology and evolution have neglected this issue [15] , [16] , [31] , such that it currently remains unknown whether modularity is simply a by-product of distance effects on movement. 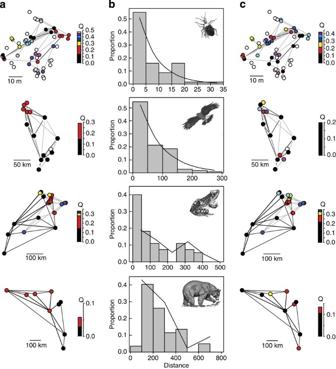Figure 1: Network modularity of individual movement and gene flow. For the four species, shown are (a) colour-coded modules (white dots reflect patch isolates with no movement) that arise when distance effects are not accounted for in module detection, (b) histograms of movement and genetic covariance along with the ‘deterrence’ function (black line) used for each species and (c) modules identified when distance effects are accounted for in module detection. Colour scales show the decomposition of module contributions to landscape modularity,Q, with colours identifying modules shown on the networks. Dot position reflects geographic location of patches. Figure 1: Network modularity of individual movement and gene flow. For the four species, shown are ( a ) colour-coded modules (white dots reflect patch isolates with no movement) that arise when distance effects are not accounted for in module detection, ( b ) histograms of movement and genetic covariance along with the ‘deterrence’ function (black line) used for each species and ( c ) modules identified when distance effects are accounted for in module detection. Colour scales show the decomposition of module contributions to landscape modularity, Q , with colours identifying modules shown on the networks. Dot position reflects geographic location of patches. Full size image To address this crucial issue, we altered the modularity function to account for geographic distance effects. Recently, modularity analysis for social network data was extended to account for distance effects [32] . We applied this general approach for each of the spatial networks, extending it to reflect metapopulation theory for connectivity [33] , [34] and potential directionality in movement. This formulation identifies whether modularity remains after accounting for dispersal kernels or isolation-by-distance in gene flow [35] . After accommodating space modularity remained, although the modules identified changed ( Fig. 1c ). Significance tests suggested that for snail kites, the observed modularity could be explained by distance effects alone (that is, movement within versus between modules was no longer statistically significant after accommodating space), whereas distance could not fully explain modularity in the other two examples where modularity was detected (significant modularity remained; Supplementary Table S1 ). Modularity and patch connectivity In modular networks, individual patches may have fundamentally different impacts on connectivity within and between modules. Guimera and Amaral [36] argued that in such networks, the universal roles of nodes (patches) can be described by their relative within-module importance or the importance of a patch to connectivity within its module compared with other patches within the same module and their ‘participation coefficient’ or the extent to which a patch is connected to all modules in a network. For each network, we assessed the relative importance of patches to connectivity by contrasting patch strength (the total observed movement or gene flow for patch i, w i ) that ignores modularity to similar measures that incorporate modularity based on the within-module strength and participation coefficient for each patch. We found that in each example, patches that tended to have high participation coefficients tended to have low within-module strength ( Fig. 2a–c ), emphasizing that patches rarely had important roles for connectivity both within and between modules. Furthermore, the rank importance of patches changed when incorporating modularity into our connectivity assessment ( Fig. 2d–f ). Although rank importance of patches was sometimes similar based on patch strength and within-module strength, rank importance based on participation coefficients diverged substantially. 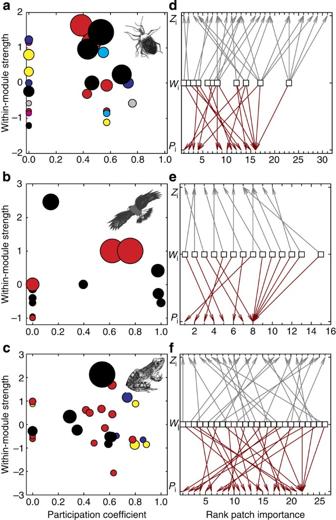Figure 2: Modularity reveals new perspectives on patch importance for connectivity and gene flow. (a–c) Within-module strength (relative importance of patches for movement within modules) and participation coefficients (the extent to which movement occurs among all modules for each patch) for each species exhibiting significant modularity, where dot size is proportional to patch strength and dot colour reflects modules shown inFig. 1a. (d–f) The changes in rank importance of patches when including modularity into assessments relative to ignoring modularity (using patch strength,wi; white squares), based on within-module strength (zi, grey arrows) and between-module participation coefficients (Pi, dark red arrows). Figure 2: Modularity reveals new perspectives on patch importance for connectivity and gene flow. ( a – c ) Within-module strength (relative importance of patches for movement within modules) and participation coefficients (the extent to which movement occurs among all modules for each patch) for each species exhibiting significant modularity, where dot size is proportional to patch strength and dot colour reflects modules shown in Fig. 1a . ( d – f ) The changes in rank importance of patches when including modularity into assessments relative to ignoring modularity (using patch strength, w i ; white squares), based on within-module strength ( z i , grey arrows) and between-module participation coefficients ( P i , dark red arrows). Full size image Modularity and metapopulation viability Although theory suggests that modularity can increase metapopulation viability, empirical assessments of such potential remain absent. We assessed how incorporating modularity may alter metapopulation viability assessments for cactus bugs. We focused on this species because it shows extinction–colonization dynamics on cactus patches that resemble metapopulation dynamics [37] . Theory suggests that the metapopulation capacity of a fragmented landscape can provide a relative measure for metapopulation viability [34] , [38] . Metapopulation capacity is defined as the leading eigenvalue of a ‘connectivity matrix’, which previously has used Euclidean distance between patches as a proxy for isolation and potential movement (Methods). However, elsewhere we have shown that statistical models developed for social networks reliably predict movements, in terms of model fit and predicting unknown linkages and improve predictions of metapopulation viability for cactus bugs compared with traditional distance-based proxies [21] . We tested for variation in predicted metapopulation capacity by fitting social network models to predict movement rates of cactus bugs, contrasting models that ignore modularity [21] to those that considered the potential for modularity [14] ( Methods ). This approach allows for altering predictions of connectivity matrices, and thus the metapopulation capacity, based on the potential for modularity in movements. Social network models provided strong support for modularity in the insect network (Bayesian Information Criterion ignoring modularity=1,143; including modularity=964; Fig. 3a ). When contrasting metapopulation capacity based on this modularity-driven, social network model to the existing theory [34] and social network models that ignored modularity [21] , we found that accounting for modularity greatly increased predictions of metapopulation capacity ( Fig. 3a ). In this context, relative patch importance (proportional contributions) to metapopulation capacity can be assessed on the basis of leading eigenvectors of the connectivity matrices [34] . Inclusion of modularity altered predictions of patch contributions to metapopulation capacity ( Fig. 3b ), suggesting that 4–5 key patches have a much greater contribution than what would be assumed when modularity is ignored. Taken together, the inclusion of modularity into metapopulation assessments was most supported by the data and had strong effects regarding the predictions of persistence of this population. 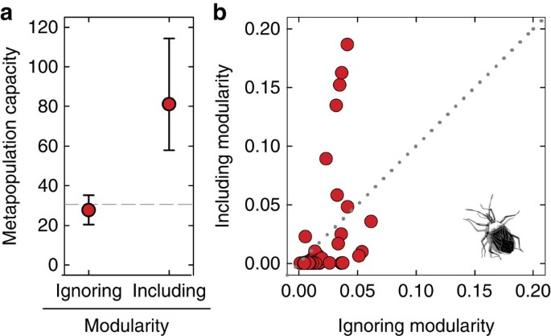Figure 3: Incorporating modularity into connectivity predictions alters conclusions on metapopulation viability for cactus bugs. (a) Estimates of metapopulation capacity on the basis of social network models that ignore the potential for modularity and include the potential for modularity (via latent space clustering parameters). The dashed line shows the theoretical prediction of metapopulation capacity using the Hanski and Ovaskainen34approach. Error bars denote variation based on the inclusion of 95% credible intervals in movement predictions. (b) Proportional patch contributions to metapopulation capacity for models that ignore the potential for modularity and include the potential for modularity. Patch contributions to metapopulation capacity are based on the squared leading eigenvectors of connectivity matrices34. Dotted diagonal line indicates no differences in proportional contributions. Figure 3: Incorporating modularity into connectivity predictions alters conclusions on metapopulation viability for cactus bugs. ( a ) Estimates of metapopulation capacity on the basis of social network models that ignore the potential for modularity and include the potential for modularity (via latent space clustering parameters). The dashed line shows the theoretical prediction of metapopulation capacity using the Hanski and Ovaskainen [34] approach. Error bars denote variation based on the inclusion of 95% credible intervals in movement predictions. ( b ) Proportional patch contributions to metapopulation capacity for models that ignore the potential for modularity and include the potential for modularity. Patch contributions to metapopulation capacity are based on the squared leading eigenvectors of connectivity matrices [34] . Dotted diagonal line indicates no differences in proportional contributions. Full size image For three of the four species considered, modularity analysis objectively identified meso-scales—above the patch and below the landscape—that are commonly hidden in biology. Only gene flow in black bears showed no significant evidence of modularity, which could be attributed to either their wide-ranging movements [27] or that modularity analysis may have limited power in small networks ( Supplementary Fig. S1 ). Fortuna et al. [15] argued that such modules represent fundamental scales for populations. Our results provide empirical support for this claim by illustrating that these scales can profoundly influence conclusions on connectivity and metapopulation viability. Moreover, our findings identify modules where other processes of ecological and evolutionary interest (for example, mate selection) are probably spatially restricted. In spatial networks, modularity can arise simply from localized movement among geographic locations when the Newman–Girvan expected value is used. Consequently, it has previously been unclear the extent to which observed modularity in spatial biology is simply driven by well-known distance effects on movement, which are frequently summarized in dispersal kernels and genetic measures of isolation-by-distance ( Fig. 1b ). Our spatial extension of this algorithm suggested that modularity occurred beyond what localized movement could explain in two of the species, the cactus bug and the bullfrog. At least two alternative hypotheses may explain this structure in cactus bugs. First, the vegetation surrounding patches (the ‘resistance’ of the matrix [39] ) may influence movement rates beyond geographic distance alone because movement of cactus bugs is influenced by vegetation height [28] in the surrounding matrix. However, this ‘matrix resistance’ hypothesis cannot, in isolation, explain modularity because replacing our null model with an effective distance based on matrix resistance (measured from vegetation height using circuit theory [39] ) still resulted in significant modularity (modularity=0.47, P <0.001). Second, aspects of patch size and quality could drive module structure beyond that captured in our null models [37] . Cactus bugs show preferential movements toward large patches [40] and the observed modules can be discriminated based on measures of patch size (MANOVA using cactus size, shape and height: Pillai’s trace=0.60, d.f.=7,48, P =0.036), providing some support for this hypothesis. For bullfrogs, genetic distances are probably influenced by both historical and contemporary ecological processes [41] ; in this instance, modularity may be confounding limited gene flow between patches with the historical process of secondary contact between allopatric lineages. Bullfrogs in Ontario represent two distinct postglacial lineages, whose distribution is very similar to that represented by the observed modules [42] after the effects of distance are removed ( Fig. 1c ). Additional effort to remove historical influences on the genetic signals of modularity should be explored, particularly, when the geographic scale of the study far exceeds the scale of ecological dispersal. In the northeastern populations, we observed spatial heterogeneity in modularity ( Fig. 1c ) that could reflect a pattern of finer-scale disequilibrium than what was described previously based on patterns of isolation-by-distance [24] . Fine-scale modularity among bullfrog populations may be driven more by habitat characteristics and the degree of aquatic connectivity than by distance. Future efforts to interpret the effect of these characteristics on movement and gene flow and incorporate these factors as a null model in modularity analysis, similar to that used for the cactus bug, may shed light on this issue. In the observed networks, key patches were generally important for either within-module connectivity or between-module connectivity—but not both. Within-module connectivity is probably relevant for facilitating colonization and rescue effects [19] and in altering the rate of genetic drift and local adaptation. Between-module connectivity may be critical for long-term metapopulation persistence and the maintenance of genetic diversity via rare dispersal events. For example, patch removal simulation experiments for the cactus bug network suggest that participation coefficients better explain changes in metapopulation capacity than do within-module strength of patches ( Supplementary Fig. S2 ). Although there are dozens of metrics that are aimed to assess both genetic and demographic connectivity at the patch and landscape scale [21] , [33] , [43] , [44] , [45] , current approaches ignore module structure. These results suggest that such metrics may be misleading when modularity occurs. Consequently, if the potential for modularity is not considered, connectivity conservation that aims to prioritize patches may incorrectly prioritize key areas, reducing the effectiveness of conservation strategies. Modularity is frequently hypothesized to be important for the stability and persistence of a wide range of networks [19] , [46] , [47] , [48] . Here, we found that inclusion of modularity into connectivity matrices via social network models substantially increased predictions of metapopulation capacity, a common index of metapopulation viability [34] , [38] . Identifying the mechanisms driving the influence of modularity on metapopulation dynamics, such as heightened rescue effects within modules due to redundant linkages [19] or asynchronous dynamics between modules [49] , will be essential for understanding how to manage and conserve populations exhibiting modularity. Modularity in populations is relevant to existing ideas in landscape ecology [50] , [51] , [52] , metapopulation biology [38] , [53] , [54] , [55] , [56] and genetics [23] , [57] , yet the concept has novel utility for identifying critical scales in connectivity for several reasons. First and foremost, module identification is an outcome rather than an input: the presence, number, strength and location of modules are unknown variables that are estimated from the data. The detection of genetic modularity is in this way different than Bayesian clustering approaches [57] that identify the most likely membership of genotypes to an a priori defined number of clusters. Second, as we show here, modularity analysis can accommodate frequent problems that currently exist in spatial analysis and are often ignored in existing spatial biology theory, such as redundancy in connectivity (beyond pair-wise comparisons), non-stationarity in ecological processes (that is, spatial trends) and anisotropy. Third, modularity can reveal spatial structure independent of geographic distance effects, thereby allowing for assessments to understand the relative contribution of isolation-by-distance and other factors to the functional aggregation of populations. Finally, other null models that impose constraints on module identification can be accommodated in a straightforward manner, such as distance between patches, matrix resistance or population density. Although modularity analysis has several advantages over existing approaches for identifying relevant spatial scales for connectivity of populations, there have been some recent criticisms of this approach in the network sciences. First, the approaches we show assume no overlap among modules (that is, it is a ‘hard’ partition) [12] . Nonetheless, overlapping modules have been considered (and observed) in other types of networks. Second, there is a known ‘resolution limit’ to modularity analysis [58] . Such resolution limits can, however, be minimized by adjusting null models to reflect biologically relevant processes, such as localized movement [12] . Third, modularity analysis often suffers from what has been termed ‘degeneracy’: when several possible module assignments provide nearly identical modularity values [59] . We note that such degeneracy could be accommodated through the use of ensemble predictions [60] of module assignments, which may also better acknowledge uncertainties in module identification. We argue that modularity probably occurs in most spatially structured populations. The concept of modularity provides a vehicle for objectively moving beyond the patch paradigm in ecology that dates back to the application of island biogeography to terrestrial systems [11] . It offers a complementary means of evaluating the appropriate scale of population genetic structure [57] and genetic connectivity [23] , and we expect it will improve our understanding of connectivity and population biology in a changing world. Focal species We analysed individual movement data from mark-recapture studies for two species: the cactus bug and the Everglades snail kite [21] . We analysed movement data of cactus bugs among 56 prickly pear cactus ( Opuntia humifusa) patches. For the snail kite, we analysed within-breeding season movements among 15 wetlands in peninsular Florida. For both species, we used a weighted, directed adjacency matrix, A , to assess modularity, where A ij represents the number of observed movements from i to j . We analysed population genetic data for two species: the bullfrog and the Florida black bear. We reanalysed the genetic data (seven microsatellite loci) from 753 bullfrogs sampled at 26 wetlands in eastern Ontario, Canada [24] . We also reanalysed genetic data from Florida black bear populations [25] , which included 12 microsatellite loci from 339 bears sampled at 9 core habitat areas in Florida. For both species, we constructed a spatial network of genetic similarity where A ij is a weighted, undirected matrix of genetic covariance [15] , [61] . These methods reduce A ij between all samples to those best explained by the conditional genetic covariance among all populations considered simultaneously. Modularity analysis A powerful approach to identifying modules comes from statistical physics and social sciences, where interest is in detecting ‘communities’ in social networks. This approach defines modularity, Q , as: where m is the total number of possible links in an undirected network, A ij is the element of the adjacency matrix that describes movement/gene flow between patches i and j , P ij is an expected value and δ ( C i , C j ) is an indicator matrix that is equal to one if i and j are members of the same module and zero otherwise [30] . We used the common, Newman–Girvan [30] expected value of w i w j /2 m to calculate Q ( Q ng hereafter), where w is the patch strength ( ) [12] . This expected value is useful in that both the strength distribution and the total amount of observed (or potential) movement on the network are conserved ( ); however, it also implicitly assumes an equal likelihood of movement among resource patches regardless of spatial location [32] (see below for relaxing this assumption). To accommodate directional movement (for example, immigration≠emigration for patches i, j), we set P ij = w i-out w j-in / w , where w i-out is the emigration rate for patch i and w j-in is the immigration rate for patch j [12] . Here, P ij accounts for immigration and emigration rates between patches, such that it identifies modularity structure that arises beyond what is expected based on patch-specific immigration and emigration rates. Because of the additive nature of the modularity function, the contributions of each module to Q can readily be assessed by summing the elements of equation 1 for each module detected ( Fig. 1 ). We used a simulated annealing algorithm to maximize the modularity function by iteratively searching for δ ( C i , C j ) that maximizes Q [36] and generalized linear models to assess significance of observed modules. Generalized linear models (GLMs) assess significance by comparing the amount of movement within modules to the amount of movement between modules [62] , thereby addressing the question: is there a significant variation in movement within versus among identified modules? In the Supplementary Methods , we contrast this approach with randomization tests based on known modules and find that GLMs are more powerful, particularly on small networks ( Supplementary Fig. S1 ). Based on these simulation results, we used Poisson GLMs for assessing the significance of identified modules for mark-recapture data and used zero-adjusted gamma GLMs for assessing significance in genetics data, where A ij included continuous values ≥0 ( Supplementary Table S1 ). Although the expected value for the modularity function is widely applied, it may be limited for applications in spatial biology because movement probabilities and gene flow of species decline, often exponentially, with distance. Recently, the expected value, P ij , has been altered to account for geographic effects in social networks when calculating Q ( Q spa hereafter) [32] : where f ( d ij ) is a ‘deterrence’ function that in this case describes variation in movement as a function of distance, d , between patches: This function is a non-parametric, data-driven function describing the probability of movement between i and j , given the distance between patches (note that ). We used this function for bullfrogs and black bears because we had no a priori expectation for parametric relationships to explain A ij as a function of distance. When using this deterrence function, distances must be binned for determining movements within distance categories. We systematically altered the bin width and then used the bin width with the highest observed Q spa ( Supplementary Fig. S3 ). For cactus bugs and snail kites, we extended the approach as: where 1/ α is the mean dispersal distance observed. This extension captures assumptions from metapopulation theory and does not require binning of empirical data (but note that we must add a scaling constant to equation 2 to satisfy ). Directed movements were accommodated in equation 2 as P ij = w i-out w j-in f ( d ij ). Consequently, directionality is captured through the incorporation of patch-specific immigration/emigration rates, rather than altering the effective distance between patches. Note that d ij could be replaced with measures of effective distance that incorporate effects of the structure of the surrounding environment (that is, the ‘matrix’), such as resistance distances or least-cost distances [39] . For cactus bugs, we considered vegetation height as a relevant aspect of matrix structure that can influence bug movement [28] and calculated resistance distances between all patches i and j (based on an interpolated resistance map of 106 vegetation height measurements and using circuit theory to estimate resistance distances [39] ). We then altered equation 4 using resistance distance to ask if modularity remained beyond what would be expected based on the surrounding matrix. Patch importance and modularity In modular networks, connectivity can vary within versus between modules. We assessed these different connectivity roles of patches using two key metrics: within-module strength and participation coefficient [36] . Within-module strength assesses the relative importance of a patch to connectivity within modules compared with other patches within the same module: where w ig is the amount of movement observed for patch i within its module g. The participation coefficient is: where N m is the number of modules in the network. P i will be zero if all movement is within the module of patch i and will approach one when movement is uniformly distributed among all modules in the network. However, because the maximum value of P i will depend on the number of modules observed (where P max =1–1/ N m ), we scale P i by dividing by P max , such that it ranges 0–1 for all networks. With these metrics, we ask whether patch prioritization differs when acknowledging modularity. We contrasted within-module strength and participation coefficient to patch strength, w i , because this measure is the most direct analogue when ignoring modularity to these modularity metrics. Thus, rankings based on patch strength prioritize patches associated with the greatest amounts of movement in the landscape, within-module strength rankings prioritize patches with the greatest amounts of movement within modules, and rankings based on the participation coefficient prioritize patches that connect modules in the landscape. Patch isolates (no observed movement) were not considered because z i is undefined. See Supplementary Figs S4–S7 for comparisons to other connectivity metrics. Modularity and metapopulation capacity Community detection uses the observed adjacency matrix, A , to interpret if modularity emerges in networks. However, a distinct and complementary approach is to ask how predictions of A change if we treat modules as a covariate in making predictions for A ij . Recently, statistical social network models have been extended to formally consider clustering (approximate modularity) in the modelling process, termed ‘latent position cluster models’ [14] . These models begin with describing a ‘latent space’, l i , for patch connectivity on networks. In the context of landscape connectivity, latent space models leverage observed similarities in movements within networks to predict A ij based on an unobservable or latent ‘connectivity space’ [21] . We modelled the probability of observed movement between patches, y ij , as a Bernoulli distribution with a mean, p ij , and included distance, d ij , between patches (pair-wise distances) as the only fixed covariate in the model. We used a Euclidean distance measure based on similarities of between-patch movements to estimate latent connectivity space, such that our model formulation is: where y ij is the observed presence or absence of a link (movement) between patches i and j, α is an intercept, β is the coefficient for distance and the latent space is: where K is the number of dimensions in the Euclidean latent space (we set K =2) [63] , [64] . This formulation of latent space is inherently symmetrical [64] . Previously, we have shown that this latent space model accurately predicts cactus bug movements [21] . Here we extend this approach by assuming that the latent space parameters l i emerge from a finite mixture of multivariate normal distributions of different groups, G , which can have different means, μ , and variances, σ 2 : where λ g is the probability that patch i belongs to module g, k is the number of latent space dimensions and I is an identity matrix [14] . We fit these models via Markov Chain Monte Carlo. Importantly, for fitting this model, one must a priori pick G , unlike the modularity optimizations we have considered. Handcock et al. [14] recommended that the choice of G be determined using a variant of Bayesian Information Criterion (BIC) developed for this model. We considered G ranging from 1 to 7 and selected the model with the lowest BIC. We followed recommendations for prior distributions and hyperparameters in this model formulation [14] . We then compared predictions when assuming no modularity ( G =1) to predictions that assume modularity ( G >1). We assessed metapopulation capacity of the cactus bug network using the conventional approach in metapopulation biology by calculating the leading eigenvalue of the ‘connectivity matrix’, M =S i S j (exp(- αd ij )) (ref. 34 ), where S i is the size of patch i. We then replaced exp(- αd ij ) with the predicted A ij from the social network model [21] that assumes no modularity ( G =1) and A ij from the best-fitting model that captured modularity ( G =5). We incorporated uncertainty in predictions of metapopulation capacity from the network models based on 200 samples of the posterior distributions of the model predictions. We estimated the relative patch importance to metapopulation capacity by squaring the elements of the leading eigenvectors of the connectivity matrices [34] . For each model, these importance values sum to one and describe the relative contribution of each patch to the predicted metapopulation capacity [34] . Finally, we used latent position cluster models coupled with a patch removal experiment to examine if the roles of within-module strength and participation coefficient of patches have differential influences on predicted metapopulation capacity. Using the best-fitting latent position cluster model, we removed each patch from the network one at a time and the metapopulation capacity was calculated. We then used two general linear models to correlate predicted metapopulation capacity with the within-module patch strength and participation coefficient of the removed patch, calculated from modules identified with both Qng and Qspa ( Supplementary Fig. S2 ). How to cite this article: Fletcher, R. J. et al. Network modularity reveals critical scales for connectivity in ecology and evolution. Nat. Commun. 4:2572 doi: 10.1038/ncomms3572 (2013).